Generation of a ciliary margin-like stem cell niche from self-organizing human retinal tissue In the developing neural retina (NR), multipotent stem cells within the ciliary margin (CM) contribute to de novo retinal tissue growth. We recently reported the ability of human embryonic stem cells (hESCs) to self-organize stratified NR using a three-dimensional culture technique. Here we report the emergence of CM-like stem cell niches within human retinal tissue. First, we developed a culture method for selective NR differentiation by timed BMP4 treatment. We then found that inhibiting GSK3 and FGFR induced the transition from NR tissue to retinal pigment epithelium (RPE), and that removing this inhibition facilitated the reversion of this RPE-like tissue back to the NR fate. This step-wise induction-reversal method generated tissue aggregates with RPE at the margin of central-peripherally polarized NR. We demonstrate that the NR–RPE boundary tissue further self-organizes a niche for CM stem cells that functions to expand the NR peripherally by de novo progenitor generation. The retina is the main visual sensory tissue in mammals. Its anlage, the optic cup, is derived from the rostral diencephalon and is composed of the inner and outer walls—the neural retina (NR) and retinal pigment epithelium (RPE), respectively [1] , [2] . Mammalian NR is known to possess a low regenerative capacity, and spontaneous tissue recovery hardly occurs following substantial damage caused by trauma or degenerative diseases. This stands in sharp contrast to the newt NR, for instance, which can fully regenerate from neighbouring RPE even after total resection (reviewed in refs 3 , 4 ). In vertebrate retinogenesis, the NR has two different groups of progenitors present in distinct locations. During early retinal development, epithelial progenitors are widely present in the NR epithelium and function to generate photoreceptors and other types of retinal neurons [5] . Their differentiation capacity gradually changes as retinogenesis proceeds; they have a tendency to produce ganglion cells and cones at early stages, and then rods and bipolar cells at late stages [6] , [7] . Like cortical progenitors, these NR progenitors show the radial glia-like morphology with thin apical and basal processes, characteristic of neuroepithelial progenitors, and they undergo interkinetic nuclear migration during mitotic cycles [8] , [9] . (Hereafter, these progenitors are referred to as ‘NR progenitors’). Another kind of progenitor is located at the peripheral margin of the NR, the ciliary margin (CM) [5] , [10] , [11] . The teleost (fish) eye contains an active stem cell system in the CM zone (also called circumferential germinal zone) that contributes to NR expansion by de novo generation of the tissue even in adulthood [12] . This type of stem cell robustly self-renews and gives rise to all NR cell types in the extending NR periphery, unlike the nonmarginal-NR progenitor, whose developmental competence gradually becomes confined to the generation of limited cell types during retinogenesis as mentioned above. In the chick embryo, the stem cell system at the CM also plays an active role during eye development, and stem cells isolated from this region can form NR tissue in floating aggregate culture [13] . The mammalian foetal eye also contains a peripheral NR zone resembling the chick embryonic CM in molecular marker expression, and this zone contains a substantial number of stem cells [10] , [14] , [15] (Hereafter, these cells are referred to as ‘CM stem cells’). The presence of a small number of retinal stem cells at the ciliary region in the adult mammalian eye has also been reported [16] , [17] , [18] , [19] , [20] , although the extent of their in vivo contribution to the maintenance and regeneration of adult retinal tissue remains elusive. Recent advancement in stem cell research has enabled in vitro differentiation of retinal progenitors and their derivatives from pluripotent stem cells [21] , [22] , [23] , [24] , [25] , [26] , [27] , [28] , [29] . Moreover, mouse and human embryonic stem cells (hESC) aggregate have been shown to possess the potential to self-form optic cups in three-dimensional (3D) culture when retinal differentiation efficiency is sufficiently high [30] , [31] , [32] . Notably, the ESC-derived NR self-organizes the formation of multiple retinal layers reminiscent of the postnatal retina. NR progenitors in this culture exhibit radial glia-like epithelial morphology, frequently proliferate with interkinetic nuclear migration and give birth to photoreceptors and other retinal neurons in a stage-dependent manner [30] , [32] , a process which largely recapitulates the activity of NR progenitors in vivo . Moreover, a recent report using mouse ES cells showed that self-forming NR tissue can give rise to functional photoreceptors capable of light response after grafting in the murine eye [33] . In the self-organized optic cup, the boundary domain between NR and RPE, called the hinge domain, contains cells with a morphology distinct from that of NR and RPE cells. However, whether CM-type stem cells are generated at this region in long-term culture has remained unexplored. In the present study, we have uncovered the formation of CM-like zones in self-organizing retinal culture. First, we made substantial improvements to the 3D culture method of hESCs for promoting retinal differentiation. As reported previously, the formation of optic cup in hESC culture is less frequent (~10% of aggregates) [32] than in mouse ESC culture. Its efficacy is also influenced by minute changes in culture conditions. In particular, our previous culture included Matrigel, a crude extract of extracellular matrix from mouse EHS sarcoma cells, for promotion of retinal differentiation and epithelialization [32] . The use of Matrigel is problematic because this undefined extract shows substantial batch-to-batch differences in promoting retinal differentiation. Furthermore, the use of animal-derived matrix proteins is also unfavourable from the viewpoint of future clinical applications. Therefore, we established culture conditions for inducing selective retinal differentiation without the use of Matrigel. Using this new 3D culture technique, we further developed a two-step method that allows a reproducible formation of NR–RPE junctions to generate CM-like zones. Combining these new methods, we demonstrate that CM-like zones self-organize in vitro and function as growth zones in the periphery of hESC-derived NR. Highly selective self-formation of NR with BMP treatment We observed in a separate study of cortical self-organization that hESC aggregates selectively differentiated into Foxg1 + telencephalic neuroepithelium when cultured in growth factor-free chemically defined medium (gfCDM) without Matrigel ( Fig. 1a ). While retinal differentiation was rarely seen under these conditions, we reasoned that the addition of certain signalling molecules to the medium might cause a shift of positional information from the telencephalic to the retinal direction, given the proximity of their anlages in the embryonic brain. 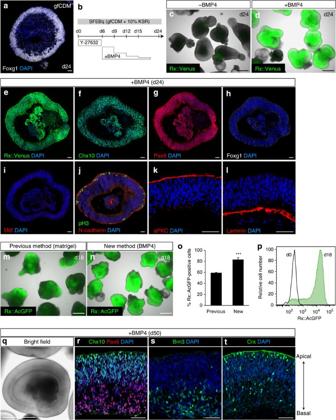Figure 1: Selective NR generation from hESC without using Matrigel. (a) Selective generation of Foxg1+telencephalic neuroectoderm (day 24) in 3D hESC culture using gfCDM without Matrigel and BMP4. Foxg1 (white) and nuclear staining with DAPI (blue). (b) Timing of BMP4 treatment. BMP4 (1.5 nM) was added to medium on day 6, while its concentration was diluted into half by half medium change on days 9, 12 and 15. (c,d) Induction ofRx::Venus by transient BMP4 treatment (d;c, untreated control) in hESC aggregates. (e–l) Immunostaining of NR tissue (day 24) generated by the improved culture method with antibodies for Venus (e), Chx10 (f), Pax6 (g), Foxg1 (h; no substantial expression), Mitf (i; no substantial expression), pH3 (j; green), N-cadherin (j; red), aPKC (k; note the strong expression on the surface of spheroid) and Laminin (l). Blue, nuclear staining with DAPI. (m–p) Comparison ofRx::AcGFP-inducing efficiency between our previous (m) and improved (new) (n) methods. (o) Percentage of AcGFP+cells in each culture on day 18 analyzed by FACS. Data represent mean±s.e.m. of three independent experiments (each experiment with 24 aggregates). ***P<0.001. Student’st-test. Representative FACS patterns for day 18 culture by the present method (green) and control undifferentiatedRx::AcGFP hESCs (day 0; black) are shown inp. (q–t) Stratified NR tissue generated by the improved method. (q) Bright field view showing the formation of continuously thick NR (day 50). (r–t) Pax6 (r; red) and Brn3 (s) were expressed in the cell layer on the basal side (ganglion cells), while Chx10+progenitors (r; green) were located in the apical layer. NR at this stage contained moderate numbers of Crx+photoreceptor precursors (t) both on the apical and basal sides. Scale bars, 500 μm (c,d,m,n,q) and 50 μm (a,e–l,r–t). See alsoSupplementary Fig. 1. Figure 1: Selective NR generation from hESC without using Matrigel. ( a ) Selective generation of Foxg1 + telencephalic neuroectoderm (day 24) in 3D hESC culture using gfCDM without Matrigel and BMP4. Foxg1 (white) and nuclear staining with DAPI (blue). ( b ) Timing of BMP4 treatment. BMP4 (1.5 nM) was added to medium on day 6, while its concentration was diluted into half by half medium change on days 9, 12 and 15. ( c , d ) Induction of Rx:: Venus by transient BMP4 treatment ( d ; c , untreated control) in hESC aggregates. ( e – l ) Immunostaining of NR tissue (day 24) generated by the improved culture method with antibodies for Venus ( e ), Chx10 ( f ), Pax6 ( g ), Foxg1 ( h ; no substantial expression), Mitf ( i ; no substantial expression), pH3 ( j ; green), N-cadherin ( j ; red), aPKC ( k ; note the strong expression on the surface of spheroid) and Laminin ( l ). Blue, nuclear staining with DAPI. ( m – p ) Comparison of Rx:: AcGFP-inducing efficiency between our previous ( m ) and improved (new) ( n ) methods. ( o ) Percentage of AcGFP + cells in each culture on day 18 analyzed by FACS. Data represent mean±s.e.m. of three independent experiments (each experiment with 24 aggregates). *** P <0.001. Student’s t -test. Representative FACS patterns for day 18 culture by the present method (green) and control undifferentiated Rx:: AcGFP hESCs (day 0; black) are shown in p . ( q – t ) Stratified NR tissue generated by the improved method. ( q ) Bright field view showing the formation of continuously thick NR (day 50). ( r – t ) Pax6 ( r ; red) and Brn3 ( s ) were expressed in the cell layer on the basal side (ganglion cells), while Chx10 + progenitors ( r ; green) were located in the apical layer. NR at this stage contained moderate numbers of Crx + photoreceptor precursors ( t ) both on the apical and basal sides. Scale bars, 500 μm ( c , d , m , n , q ) and 50 μm ( a , e – l , r – t ). See also Supplementary Fig. 1 . Full size image We therefore examined the effects of several candidate signals that are known to affect retinal differentiation (see Methods for details). Using Venus-knock-in reporter hESCs for Rx (retinal marker) [32] , [34] expression, we observed that a transient treatment of hESC aggregates with a low concentration of Bone morphogenetic protein-4 (BMP4; starting at 1.5 nM on day 6 and subject to half-dilution every 3rd day) dramatically increased Rx:: Venus expression ( Fig. 1b–d ; >95% of hESC aggregates contained Venus + epithelium on day 24; the timed application is important, since BMP4 treatment from day 0 did not promote retinal nor neural differentiation). Most of the BMP4-induced Venus + epithelium was positive for Rx, Chx10 (ref. 35 ), Pax6 and Sox2 (neural retinal marker), and negative for Foxg1 and the RPE marker Mitf ( Fig. 1e–i and Supplementary Fig. 1a ), reminiscent of the expression profile of NR epithelium. This NR epithelium reproducibly contained phospho-Histone H3 + mitotic cells on the outer surface, which accumulated the apical marker aPKC ( Fig. 1j,k ; also showing strong N-cadherin localization there). The basement membrane positive for Laminin and Collagen IV ( Fig. 1l and Supplementary Fig. 1b ) spontaneously formed on the luminal side in this culture without the addition of exogenous matrix proteins such as Matrigel. The induction efficacy of Rx:: AcGFP (a separately derived reporter line) exceeded 80% at the cellular level ( Fig. 1m–p and Supplementary Fig. 1c,d ), which is substantially higher than the efficiency seen in previous Matrigel-based cultures [32] . Thus, our new culture method enabled efficient generation of human NR epithelium under nearly defined conditions except for the inclusion of a commonly used knockout serum replacement (KSR) additive. On day 50, the epithelia were continuous and thick ( Fig. 1q ), and contained cells expressing NR cell type-specific markers such as Brn3 and Pax6 for ganglion cells ( Fig. 1r,s ), Crx for photoreceptors ( Fig. 1t ), Calretinin for ganglion cells and interneurons ( Supplementary Fig. 1e ), and Ptf1a for interneurons ( Supplementary Fig. 1f ) in addition to Chx10 + NR progenitors ( Fig. 1r ). Taken together, these observations show that selective NR differentiation from hESCs without the use of Matrigel is enabled simply by a transient early BMP4 treatment. The strong promotion of NR differentiation by BMP4 treatment was rather unexpected, since the inductive role of BMP signals is known for RPE specification [36] but not for early NR differentiation. The BMP4 treatment was transiently given at the early phase of culture, while the NR–RPE specification occurs later around day 18–20 and optic cup formation around day 24 (ref. 32 ). Therefore, we speculate that this effect could be relevant to the role of BMP signals in early forebrain patterning (this point is discussed later). Generation of RPE next to NR by induction-reversal culture In the embryonic eye, the CM arises from the hinge region joining the NR and RPE. Although the BMP-induced retinal differentiation culture was highly efficient, the retinal epithelium mostly consisted of NR ( Fig. 1f ), lacking RPE or a NR–RPE junction ( Fig. 1i ). This is consistent with the idea that NR differentiation is the default direction of retinal differentiation in ESC culture [30] . Our previous hESC study [32] showed that RPE differentiation could be induced from hESC-derived retinal epithelium by treating with canonical Wnt signals from day 18 (RPE-inducing roles of Wnt signals in vivo are also reported and discussed in refs 37 , 38 , 39 , 40 ). Conversely, FGF signals have been shown to promote NR differentiation and suppress RPE differentiation [41] , [42] . Based on these effects (summarized in Supplementary Fig. 2 ), we next sought to induce RPE differentiation in a limited domain within the hESC-derived retinal epithelium. When BMP-induced Chx10 + retinal epithelium was treated with the GSK3 inhibitor CHIR99021 (Wnt agonist) and the FGFR inhibitor SU5402 for 6 days from day 18 ( Fig. 2a , condition 2), the epithelium became thin and expressed Mitf but not Chx10 on day 24 (these RPE features were found in >90% of aggregates), whereas most of the nontreated epithelium ( Fig. 2a , condition 1) remained thick and Chx10 + /Mitf − ( Fig. 2b ). Rx:: Venus expression, which was initially strong on day 18, became dim in the epithelium after treatment with GSK3 and FGFR inhibitors (see below; Rx expression is much weaker in RPE than in NR). Thus, Wnt signal augmentation and FGF signal inhibition for a relatively short period was sufficient to induce RPE-type epithelium from Chx10 + NR progenitors. 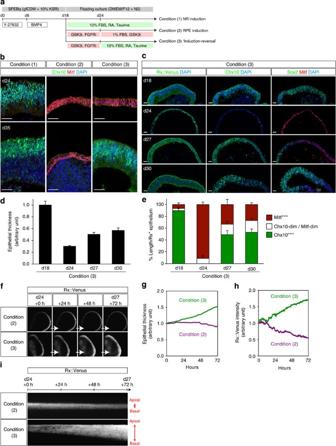Figure 2: NR–RPE conversion in induction-reversal culture. (a) Time table for three culture conditions. (b) Immunostaining of retinal epithelia cultured under conditions 1 (left), 2 (middle) and 3 (right) on day 24 (top) and day 35 (bottom). Under condition 2 on day 35, debris and mesenchymal cells were located basally under Mitf+epithelia. (c–e) Retinal epithelia cultured under condition 3 on day 18, 24, 27 and 30. (c) Immunostaining. (d) Change in epithelial thickness (fold change relative to day 18) during induction-reversal culture. Data represent mean±s.e.m. (each experiment with three representative points per aggregates (eight aggregates); each point was at the middle area of epithelial tissue). (e) Change in percentages of the length of the apical surface of Chx10-strong (green), Chx10-dim/Mitf-dim (white) or Mitf-strong (brown) epithelium in theRx::Venus+epithelium during induction-reversal culture. Data represent mean±s.e.m. (each experiment with eight aggregates). (f–i) Live-imaging analysis (f) of changes in epithelial thickness (g; fold change relative to 0 h) andRx::Venus signal intensity (h; fold change relative to 0 h; meanRx::Venus intensity in NR epithelium was shown) during induction-reversal culture. 0 h, day 24. conditions 2 and 3, top and bottom (f) or purple and green lines (g,h), respectively. Note that the increase of epithelial thickness andRx::Venus signal intensity cultured under condition 3. (i) Kymograph of live imaging data ofRx::Venus+retinal epithelia cultured under conditions 2 (top) and 3 (bottom) from day 24 to day 27. Red arrows represent apico-basal polarity. Scale bars, 50 μm (b,c). See alsoSupplementary Fig. 2. Figure 2: NR–RPE conversion in induction-reversal culture. ( a ) Time table for three culture conditions. ( b ) Immunostaining of retinal epithelia cultured under conditions 1 (left), 2 (middle) and 3 (right) on day 24 (top) and day 35 (bottom). Under condition 2 on day 35, debris and mesenchymal cells were located basally under Mitf + epithelia. ( c – e ) Retinal epithelia cultured under condition 3 on day 18, 24, 27 and 30. ( c ) Immunostaining. ( d ) Change in epithelial thickness (fold change relative to day 18) during induction-reversal culture. Data represent mean±s.e.m. (each experiment with three representative points per aggregates (eight aggregates); each point was at the middle area of epithelial tissue). ( e ) Change in percentages of the length of the apical surface of Chx10-strong (green), Chx10-dim/Mitf-dim (white) or Mitf-strong (brown) epithelium in the Rx:: Venus + epithelium during induction-reversal culture. Data represent mean±s.e.m. (each experiment with eight aggregates). ( f – i ) Live-imaging analysis ( f ) of changes in epithelial thickness ( g ; fold change relative to 0 h) and Rx:: Venus signal intensity ( h ; fold change relative to 0 h; mean Rx:: Venus intensity in NR epithelium was shown) during induction-reversal culture. 0 h, day 24. conditions 2 and 3, top and bottom ( f ) or purple and green lines ( g , h ), respectively. Note that the increase of epithelial thickness and Rx:: Venus signal intensity cultured under condition 3. ( i ) Kymograph of live imaging data of Rx:: Venus + retinal epithelia cultured under conditions 2 (top) and 3 (bottom) from day 24 to day 27. Red arrows represent apico-basal polarity. Scale bars, 50 μm ( b , c ). See also Supplementary Fig. 2 . Full size image Interestingly, the fate of the induced Mitf + epithelial cells was not irreversibly fixed even after they exhibited these molecular and morphological characteristics of RPE ( Fig. 2b ). When hESC-derived retinal epithelium was treated with CHIR99021 and SU5402 (days 18–24) and subsequently cultured in NR-differentiation medium (not containing these inhibitors) from day 24 ( Fig. 2a , condition 3), the majority of epithelium (in ~70% of aggregates) repressed Mitf expression in their major portions, regained Chx10 expression and increased the epithelial thickness ( Fig. 2b–e ). This stands in contrast to the thin Mitf1 + epithelium cultured continuously in the presence of the CHIR99021 (condition 2; Fig. 2a,b ). Live imaging analysis ( Supplementary Movies 1 and 2 , Fig. 2f–i ) showed that the recovery of the Rx:: Venus-strong thick epithelium (NR type) in the aggregates did not occur by rapid local regrowth of residual NR-type epithelium but by the transition from Rx:: Venus-dim thin epithelium (RPE type) to Rx:: Venus-strong thick epithelium. In fact, recovery of epithelial thickness and Rx:: Venus levels was already seen within the first few days after removal of GSK3 and FGFR inhibitors ( Fig. 2f–i ). This suggests that retinal differentiation, even after the appearance of early RPE features, can be reversed and redirected towards the NR fate simply by culturing the tissue in NR-differentiation medium. Hereafter, we refer to this step-wise culture (RPE induction followed by reversal to NR epithelium) as ‘induction-reversal’ culture (its possible mechanism is interpreted later in Discussion). On day 35, in contrast to NR- and RPE-inducing conditions 1 and 2 ( Fig. 3a,b ), ~40% of retinal aggregates in the induction-reversal culture (condition 3) exhibited a characteristic two-domain pattern: a large semispherical domain of continuous NR epithelium (with strong Rx:: Venus expression) with a small pigmented domain (or a few small domains) of thin and winding RPE in an adjacent location ( Fig. 3c ). This type of aggregates (two-domain aggregates, hereafter) could be easily selected (even without using microscope) for further culture ( Fig. 3d at day 60). 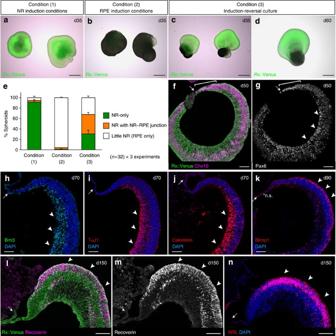Figure 3: Co-generation of NR and RPE by induction-reversal culture. (a–e) External appearance of self-formed NR and RPE structures under different conditions on day 35 (a–c,e) and day 60 (d). (a) condition 1, (b) condition 2, (c,d) condition 3. (e) Percentages of three types of aggregates. Orange corresponds to the two-domain aggregates seen inc. Data represent mean±s.e.m. (n=3 experiments, each experiment with 32 aggregates). (f–n) Immunostaining of NR tissues in the two-domain aggregates sectioned along the central-peripheral axis. (f,g) Day 50. (h–j) day 70. (k) day 90. (l–n) day 150. Arrows indicate the NR–RPE junctions (f–n). Arrowheads and brackets (f,g), the central portion abundant with Pax6+/Chx10−cells (arrowheads) and the peripheral portion preferentially containing Pax6+/Chx10+cells (bracket). Arrowheads (h–n), the central portion abundant with Brn3 (h), TuJ1 (i), Calretinin (j), Blimp1 (k), Recoverin (l,m) and NRL (n). *n.s., nonspecific staining. Scale bars, 500 μm (a–d) and 100 μm (f–n). See alsoSupplementary Fig. 3. Figure 3e shows quantitative comparison of two-domain aggregate generation (shown in orange) between conditions 1, 2 and 3 at day 35. Figure 3: Co-generation of NR and RPE by induction-reversal culture. ( a – e ) External appearance of self-formed NR and RPE structures under different conditions on day 35 ( a – c , e ) and day 60 ( d ). ( a ) condition 1, ( b ) condition 2, ( c , d ) condition 3. ( e ) Percentages of three types of aggregates. Orange corresponds to the two-domain aggregates seen in c . Data represent mean±s.e.m. ( n =3 experiments, each experiment with 32 aggregates). ( f – n ) Immunostaining of NR tissues in the two-domain aggregates sectioned along the central-peripheral axis. ( f , g ) Day 50. ( h – j ) day 70. ( k ) day 90. ( l – n ) day 150. Arrows indicate the NR–RPE junctions ( f – n ). Arrowheads and brackets ( f , g ), the central portion abundant with Pax6 + /Chx10 − cells (arrowheads) and the peripheral portion preferentially containing Pax6 + /Chx10 + cells (bracket). Arrowheads ( h – n ), the central portion abundant with Brn3 ( h ), TuJ1 ( i ), Calretinin ( j ), Blimp1 ( k ), Recoverin ( l , m ) and NRL ( n ). *n.s., nonspecific staining. Scale bars, 500 μm ( a – d ) and 100 μm ( f – n ). See also Supplementary Fig. 3 . Full size image Immunostaining on day 50 showed that the two-domain aggregate contained continuous NR epithelium positive for Rx:: Venus and Chx10 ( Fig. 3f ). Notably, the NR epithelium exhibited a gradual change in shape along the proximal-distal axis relative to RPE; the closer to RPE, the thinner the NR epithelium. In addition, molecular marker distribution exhibited an intriguing graded pattern. During in vivo development, differentiation of fate-specified retinal cells starts earlier in the central domain and is delayed in the peripheral portion [43] , [44] . For instance, Pax6 is initially expressed at high levels in all Chx10 + NR progenitors. However, as neurogenesis begins in the NR, Pax6 expression becomes attenuated in progenitors except in the peripheral domain, and becomes strong in postmitotic ganglion cells (Pax6 + /Chx10 − ) in the central domain. In hESC-derived retina, strong expression of Pax6 in Chx10 + progenitors was seen preferentially in the NR margin next to the NR–RPE junction ( Fig. 3f,g ; arrow, junction; bracket, NR margin), whereas Pax6 + /Chx10 − ganglion cells were mostly found in the nonmarginal portion of the NR ( Fig. 3g , arrowheads). Consistent with this idea, the nonmarginal NR portion also contained more cells positive for the postmitotic neuronal markers Brn3, TuJ1 and Calretinin ( Fig. 3h–j ) than the marginal NR portion. Moreover, differentiated photoreceptors marked by Blimp1, Recoverin or NRL ( Fig. 3k–n ; Supplementary Fig. 3a,b , see Methods) were preferentially located in the NR epithelium at a distance from the NR–RPE junction, indicating that differentiation of NR is more advanced in the nonmarginal NR portion (hereafter, the ‘marginal’–‘nonmarginal’ axis is referred to as the peripheral-central axis, in analogy to the in vivo situation). Collectively, these observations demonstrate that our 3D hESC culture, in which selective retinal differentiation and the induction-reversal process are combined, enables the adjacent formation of NR and RPE tissues. In the two-domain retinal structure generated by this culture, the continuity and integrity of NR epithelium was more efficiently maintained in long-term culture. While the aggregates carrying only NR (those generated typically in condition 1) tended to be discontinuous and break into small rosettes in culture beyond day 60 ( Supplementary Fig. 3c , left), the NR in the two-domain aggregates (condition 3) more frequently contained continuous epithelial structures ( Supplementary Fig. 3c,d ). The continuous NR exhibited a graded regional difference (or polarity) along the central-peripheral axis. In addition, this NR margin that was adjacent to RPE had a characteristic ‘tapering’ morphology of epithelium, which is also seen in the periphery of the foetal NR [10] , [45] . Therefore, we became intrigued by the possibility that this NR–RPE junction may have some similarity to the embryonic CM, and thus examined this region for the expression of CM-characteristic molecular markers. Expression of CM markers in the self-organized retina In hESC-derived retina ( Fig. 4a–h ; day 63), the NR–RPE junctional region expressed a set of regional markers characteristic for the embryonic CM in a complex but spatially controlled manner (refs 45 , 46 , 47 , 48 , 49 and Supplementary Fig. 4a ). The thin Mitf + epithelium ( Fig. 4a ) near the junction expressed the ciliary epithelium marker Aquaporin1 (Aqp1; Fig. 4b ) and the CM marker Otx1 ( Fig. 4c ). In contrast, the CM markers Zic1, Rdh10 and SSEA1 ( Fig. 4d,f,g and Supplementary Fig. 4b–d ), as well as the NR marker Sox2 ( Fig. 4f ) were expressed only in the Chx10 + domain ( Fig. 4e ). Interestingly, Aqp1 and Otx1 were expressed across the junction, that is, in both Mitf + and Chx10 + epithelia ( Fig. 4b,c ). 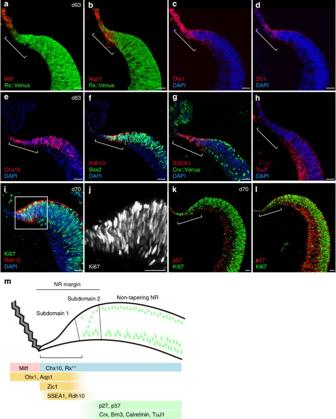Figure 4: Subdomain-specific expression of CM markers in the NR margin. (a–l) Immunostaining analysis of CM-related markers in the NR margin of hESC-derived retina generated by the induction-reversal method: Mitf (a), Aquaporin1 (b), Otx1 (c), Zic1 (d),Rx::Venus (a,b), Chx10 (e), Sox2 (f), Rdh10 (f,i), SSEA1 (g),Crx::Venus (g; strong expression in photoreceptor precursors and week expression in early RPE), TuJ1 (h), Ki67 (i–l), p57 (k) and p27 (l). (a–h) Day 63. (i–l) day 70. Bracket represents CM-like zone. (j) High magnification of the boxed area ini. (m) Schematic of marker localization in the CM-like zone around the NR–RPE junction. Scale bars, 50 μm (a–l). See alsoSupplementary Fig. 4. Figure 4: Subdomain-specific expression of CM markers in the NR margin. ( a – l ) Immunostaining analysis of CM-related markers in the NR margin of hESC-derived retina generated by the induction-reversal method: Mitf ( a ), Aquaporin1 ( b ), Otx1 ( c ), Zic1 ( d ), Rx:: Venus ( a , b ), Chx10 ( e ), Sox2 ( f ), Rdh10 ( f , i ), SSEA1 ( g ), Crx:: Venus ( g ; strong expression in photoreceptor precursors and week expression in early RPE), TuJ1 ( h ), Ki67 ( i – l ), p57 ( k ) and p27 ( l ). ( a – h ) Day 63. ( i – l ) day 70. Bracket represents CM-like zone. ( j ) High magnification of the boxed area in i . ( m ) Schematic of marker localization in the CM-like zone around the NR–RPE junction. Scale bars, 50 μm ( a – l ). See also Supplementary Fig. 4 . Full size image The tapered NR epithelium, showing a gradual increase in thickness going distally from the thin Mitf + epithelium, appeared to have two subdomains. The Chx10 + NR margin directly next to the thin Mitf + epithelium (hereafter, subdomain 1 (sd 1)) expressed CM markers such as Otx1, SSEA1, Zic1 and Rdh10, but not fate-specific NR cell markers such as TuJ1 and Crx:: Venus ( Fig. 4c–h and Supplementary Fig. 4b–d ; brackets). In contrast, the region of the tapering NR epithelium that lies distally to sd 1 (sd 2, hereafter) contained not only Chx10 + and Sox2 + progenitors ( Fig. 4e,f ), but also the fate-specific NR cell markers ( Fig. 4g,h ), particularly on its distal side. Conversely, no expression of Otx1, SSEA1, Zic1 and Rdh10 was observed in this region. While both sd 1 and sd 2 in the tapering proximal NR contained Ki67 + mitotic cells ( Fig. 4i,j ), the two subdomains differed in the expression of CDK inhibitors (p21, p27 and p57), which positively control cell cycle exit [50] , [51] ; sd 1 was mostly negative for p27 and p57, while sd 2 contained substantial numbers of cells positive for these CDK inhibitors ( Fig. 4k,l ). Expression of p21 was observed in neither subdomain ( Supplementary Fig. 4e–g ). Together, these findings (summarized in Fig. 4m ) indicate that the tapered epithelium portion adjacent to the NR–RPE junction, sd 1, has an expression profile resembling that of the in vivo CM zone. Sphere-forming progenitors from CM-like zones We next examined whether the hESC-derived CM-like region, like the foetal CM, contains sphere-forming progenitors ( Fig. 5a ). We manually dissected nonpigmented Rx:: Venus-strong tissues in the tapered NR margin (CM-like tissues, hereafter) from hESC-derived retina (day 60–85), dissociated them, and then subjected them to retinosphere culture (1,000 cells per well) [17] , [52] , [53] . For comparison, we dissected nonmarginal NR (central NR) tissues from the same aggregates. 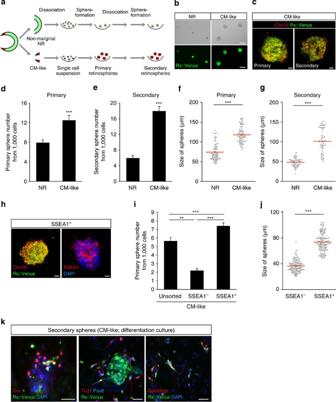Figure 5: Retinosphere formation from cells of CM-like tissues. (a) Schematic of retinosphere formation assays of cells from hESC-derived NR. (b) External appearance of primary spheres formed from dissociated cells of CM-like (right) and nonmarginal NR (left) tissues of hESC-derived NR (day 85). (c) Expression ofRx::Venus and Chx10 in primary and secondary spheres forming from dissociated cells of CM-like tissues of hESC-derived NR (day 70). (d) Number of primary spheres forming from 1,000 dissociated cells of these tissues (day 70). Data represent mean±s.e.m. of 12 experiments (each experiment with 8 samples; counted spheres, NR=759, CM-like=1,198). (e) Number of secondary spheres forming from 1,000 dissociated cells of corresponding primary spheres (formed from tissues on day 70 and cultured under sphere-forming conditions for 14 days). Data represent mean±s.e.m. of 6 experiments (each experiment with 8 samples; counted spheres, NR=286, CM-like=862). (f,g) Sizes (maximum diameters) of forming primary (f) and secondary (g) spheres. Red lines represent the mean sizes. (h) Immunostaining of retinospheres forming in dissociation suspension culture of FACS-sortedRx::Venus+SSEA1+cells from hESC-derived CM-like tissues. (i) Number of spheres forming from CM-like tissues (unsorted), MACS-purified SSEA1+cells (SSEA1+) and SSEA1−cells (SSEA1−), which were sorted from day 79 and plated at the density of 1,000 cells per well. Data represent mean±s.e.m. of 6 experiments (each experiment with 8 samples; counted spheres, unsorted=272, SSEA1−=106, SSEA1+=356). (j) Size of spheres from FACS-purifiedRx::Venus+SSEA1+cells andRx::Venus+SSEA1−cells. Red line represents the mean size. (k) Expression of fate-specific cell markers in differentiation culture of CM-like-tissue-derived secondary spheres. (d,e) ***P<0.001. Student’st-test. (i) **P<0.01. ***P<0.001. Analysis of variance followed bypost-hocTukey’s test. (f,g,j) ***P<0.001. Mann–Whitney’s test. Scale bars, 100 μm (b), 50 μm (k) and 25 μm (c,h). See alsoSupplementary Fig. 5. Figure 5: Retinosphere formation from cells of CM-like tissues. ( a ) Schematic of retinosphere formation assays of cells from hESC-derived NR. ( b ) External appearance of primary spheres formed from dissociated cells of CM-like (right) and nonmarginal NR (left) tissues of hESC-derived NR (day 85). ( c ) Expression of Rx:: Venus and Chx10 in primary and secondary spheres forming from dissociated cells of CM-like tissues of hESC-derived NR (day 70). ( d ) Number of primary spheres forming from 1,000 dissociated cells of these tissues (day 70). Data represent mean±s.e.m. of 12 experiments (each experiment with 8 samples; counted spheres, NR=759, CM-like=1,198). ( e ) Number of secondary spheres forming from 1,000 dissociated cells of corresponding primary spheres (formed from tissues on day 70 and cultured under sphere-forming conditions for 14 days). Data represent mean±s.e.m. of 6 experiments (each experiment with 8 samples; counted spheres, NR=286, CM-like=862). ( f , g ) Sizes (maximum diameters) of forming primary ( f ) and secondary ( g ) spheres. Red lines represent the mean sizes. ( h ) Immunostaining of retinospheres forming in dissociation suspension culture of FACS-sorted Rx:: Venus + SSEA1 + cells from hESC-derived CM-like tissues. ( i ) Number of spheres forming from CM-like tissues (unsorted), MACS-purified SSEA1 + cells (SSEA1 + ) and SSEA1 − cells (SSEA1 − ), which were sorted from day 79 and plated at the density of 1,000 cells per well. Data represent mean±s.e.m. of 6 experiments (each experiment with 8 samples; counted spheres, unsorted=272, SSEA1 − =106, SSEA1 + =356). ( j ) Size of spheres from FACS-purified Rx:: Venus + SSEA1 + cells and Rx:: Venus + SSEA1 − cells. Red line represents the mean size. ( k ) Expression of fate-specific cell markers in differentiation culture of CM-like-tissue-derived secondary spheres. ( d , e ) *** P <0.001. Student’s t -test. ( i ) ** P <0.01. *** P <0.001. Analysis of variance followed by post-hoc Tukey’s test. ( f , g , j ) *** P <0.001. Mann–Whitney’s test. Scale bars, 100 μm ( b ), 50 μm ( k ) and 25 μm ( c , h ). See also Supplementary Fig. 5 . Full size image While Rx:: Venus + primary retinospheres formed from both CM-like and central-NR groups ( Fig. 5b,c ; note that non-CM-type NR progenitors were also present in the central-NR tissues), the efficacy was higher with cells from CM-like tissues ( Fig. 5d and Supplementary Fig. 5a ). Secondary sphere formation (1,000 cells per well) also showed a clear difference in efficacy ( Fig. 5e ; central-NR group <CM-like group). Furthermore, the sizes of both primary and secondary spheres from CM-like tissue were significantly larger than those from central NR ( Fig. 5b,f,g and Supplementary Fig. 5b ). The majority of cells in the primary and secondary retinospheres from CM-like tissues were Chx10 + progenitors ( Fig. 5c ). These findings suggested that the CM-like tissue contains self-renewing progenitors with a robust proliferative capacity. To confirm that sd 1 cells in the CM-like tissue have the sphere-forming ability, we next examined the activity of the SSEA1 + cells purified from hESC-derived CM-like tissues ( Fig. 5h–j and Supplementary Fig. 5c,d ). SSEA1 + cells (purified by fluorescent-activated cell sorting (FACS) or magnetic-activated CS (MACS)) formed retinospheres ( Fig. 5h ) more frequently than did SSEA1 − cells ( Fig. 5i ; MACS tended to have a better cell viability than FACS; Supplementary Fig. 5d ). In addition, spheres from SSEA1 + cells were substantially larger in size than those from SSEA1 − cells ( Fig. 5j ). Although SSEA1 − cells may still have the potential to form retinospheres, these findings indicate that SSEA1 + cells play a major role in sphere formation from CM-like tissues. When cultured under differentiation conditions (adhesion culture) for 2 weeks, retinospheres from CM-like tissues (both primary and secondary) produced cells expressing fate-specific retinal cell markers such as Crx/Blimp1 (photoreceptors), TuJ1/Pax6 (ganglion cells) and Calretinin (ganglion cells and interneurons; Fig. 5k and Supplementary Fig. 5e ). The generation of fate-specific retinal cells from spheres was also observed with SSEA1-sorted cells after 2-week culture ( Supplementary Fig. 5f ), while few differentiated cells were seen initially. Taken together, these observations indicate that the NR–RPE junction zone of hESC-derived retina not only has a characteristic CM expression profile, but also contains sphere-forming progenitors resembling CM stem cells. De novo NR generation at hESC-derived CM-like zones We next investigated the progenitor dynamics at the CM-like zone of hESC-derived retina, focusing on de novo generation of NR tissue at its margin. To this end, we performed pulse-labelling experiments using nucleotide analogues (BrdU and EdU; Fig. 6 ). One-day exposure of hESC-derived retina to BrdU heavily labelled most cells in sd 1 ( Fig. 6a ) and a majority of cells in sd 2. These cells expressed the mitotic marker Ki67 ( Fig. 6a , top). When the pulse-labelled tissues were cultured without BrdU for an additional 6 days, the cells in sd 1 rarely retained BrdU labelling ( Fig. 6b , sd 1), suggesting that sd 1 mainly contains actively proliferating progenitors in which BrdU was diluted by cell division (the loss of BrdU + cells was unlikely to be caused by selective cell death, since this subdomain showed no substantial accumulation of cleaved caspase 3, a marker for apoptosis; Supplementary Fig. 6a ). 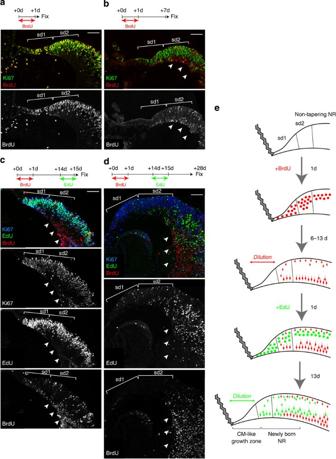Figure 6: CM-like subdomain in hESC-derived NR functioning as a growth zone. (a) Distribution of BrdU incorporation (red) after a 1-day BrdU exposure (starting at day 60). Immunostaining of Ki67, green. Note that most of the Ki67+cells in subdomain 1 (sd 1), subdomain 2 (sd 2) and central NR are positive for BrdU. (b) Distribution of BrdU-retaining cells after an additional 6-day culture without BrdU. Note that most of Ki67+cells in sd 1 and sd 2 are negative for BrdU (brackets) and most of BrdU+cells in basal side of sd 2 and central NR are negative for Ki67 (arrowheads). (c) Distribution of BrdU-retaining cells (red) pulse labelled 2 weeks before (starting at day 60) and of EdU-labelled cells (green) by exposure over the last 24 h. Note that most of the Ki67+cells in sd 1 and sd 2 are EdU+BrdU−(brackets) and most of BrdU+cells in basal side of sd 2 and central NR are negative for Ki67 (arrowheads). (d) Distribution of BrdU-retaining cells (red) pulse labelled 4 weeks ago (starting at day 60) and of EdU-labelled cells (green) pulse labelled 2 weeks ago. Note that most of Ki67+cells in sd 1 and sd 2 are negative for EdU nor BrdU (brackets) and most of BrdU+cells or EdU+cells in basal side of sd 2 and central NR are negative for Ki67 (arrowheads). (a–d) Brackets, sd 1 and sd 2. Scale bars, 100 μm (a–d). (e) Summary of results of BrdU/EdU-labelling analyses. See alsoSupplementary Fig. 6. Figure 6: CM-like subdomain in hESC-derived NR functioning as a growth zone. ( a ) Distribution of BrdU incorporation (red) after a 1-day BrdU exposure (starting at day 60). Immunostaining of Ki67, green. Note that most of the Ki67 + cells in subdomain 1 (sd 1), subdomain 2 (sd 2) and central NR are positive for BrdU. ( b ) Distribution of BrdU-retaining cells after an additional 6-day culture without BrdU. Note that most of Ki67 + cells in sd 1 and sd 2 are negative for BrdU (brackets) and most of BrdU + cells in basal side of sd 2 and central NR are negative for Ki67 (arrowheads). ( c ) Distribution of BrdU-retaining cells (red) pulse labelled 2 weeks before (starting at day 60) and of EdU-labelled cells (green) by exposure over the last 24 h. Note that most of the Ki67 + cells in sd 1 and sd 2 are EdU + BrdU − (brackets) and most of BrdU + cells in basal side of sd 2 and central NR are negative for Ki67 (arrowheads). ( d ) Distribution of BrdU-retaining cells (red) pulse labelled 4 weeks ago (starting at day 60) and of EdU-labelled cells (green) pulse labelled 2 weeks ago. Note that most of Ki67 + cells in sd 1 and sd 2 are negative for EdU nor BrdU (brackets) and most of BrdU + cells or EdU + cells in basal side of sd 2 and central NR are negative for Ki67 (arrowheads). ( a – d ) Brackets, sd 1 and sd 2. Scale bars, 100 μm ( a – d ). ( e ) Summary of results of BrdU/EdU-labelling analyses. See also Supplementary Fig. 6 . Full size image In contrast, BrdU-labelled Ki67-negative cells, representing newly born postmitotic cells, appeared in sd 2 (red cells in Fig. 6b , sd 2). Next, we cultured the tissue for 13 days after 1-day BrdU labelling and then treated with EdU for 1 day ( Fig. 6c ). In this case too, EdU uptake was seen in most Ki67 + cells in both sd 1 and sd 2. In contrast, BrdU label-retaining cells were found in the central side of sd 2, but rarely in sd 1 or the peripheral side of sd 2 ( Fig. 6c ). After the tissue was further cultured for an addition 13 days, BrdU-retaining cells were found in the thick portion of the NR but rarely in sd 1 and sd 2, while EdU-retaining cells were seen also in sd 2 ( Fig. 6d ). These EdU-retaining cells expressed fate-specific markers such as Brn3, Crx and Calretinin ( Supplementary Fig. 6b–d ). Collectively, these findings demonstrate dynamic generation and differentiation of progenitors in distinct subdomains around the CM-like zone of the hESC-derived retina ( Fig. 6e ). In sd 1, the epithelium consists mostly of actively proliferating Ki67 + cells and the nucleotide analogue labels in these cells are diluted fast by continuous cell division, suggesting that this is a place for the de novo production of progenitors from stem cells rather than a site for generation of postmitotic cells. In contrast, sd 2 have Ki67 + cells predominantly on the apical side and gradually accumulates Ki67 − postmitotic cells on the basal side as it goes farther from the NR–RPE junction, suggesting that postmitotic cells are generated in this subdomain, unlike sd 1. This idea is consistent with the observation that the CDK inhibitors p27 and p57 are expressed in sd 2 but rarely expressed in sd 1 ( Fig. 4k,l and Supplementary Fig. 4b–d ). Within sd 2, label-retaining cells gradually disappear from the peripheral to central direction during a time course of 1–4 weeks, such that cells labelled earlier are found more distally from the NR–RPE junction. Taken together with the observation that sphere-forming SSEA1 + cells are densely present in sd 1 ( Figs 4g and 5i ), these findings indicate that the hESC-derived CM-like tissue constitutes a growth zone for de novo generation of retinal progenitors at the NR–RPE boundary in self-organizing retinal culture ( Fig. 7 ). 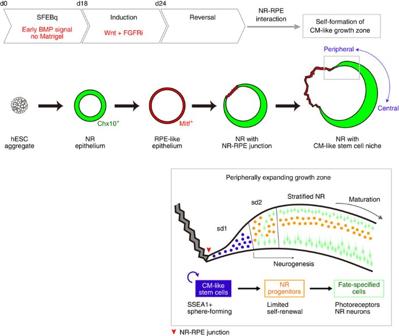Figure 7: Self-organization of growth zone with stem cell niche from hESCs. Schematic of self-organization culture of hESCs involving selective NR differentiation with transient BMP4 treatment, induction-reversal culture and self-formation of CM-like tissue at the NR–RPE boundary. Inset, schematic of a self-forming CM-like zone at the margin of hESC-derived NR with SSEA1+sphere-forming stem cells (blue), which produces NR progenitors. The CM-like growth zone functions in a similar manner with the progress zone in the developing limb, with regard to self-renewal and tissue extension. Figure 7: Self-organization of growth zone with stem cell niche from hESCs. Schematic of self-organization culture of hESCs involving selective NR differentiation with transient BMP4 treatment, induction-reversal culture and self-formation of CM-like tissue at the NR–RPE boundary. Inset, schematic of a self-forming CM-like zone at the margin of hESC-derived NR with SSEA1 + sphere-forming stem cells (blue), which produces NR progenitors. The CM-like growth zone functions in a similar manner with the progress zone in the developing limb, with regard to self-renewal and tissue extension. Full size image A long-standing question regarding the formation of the human eye is how new cells—both progenitors and postmitotic—are added to the rapidly expanding NR during foetal development. Previous studies in nonhuman model systems, have suggested that the CM of the eye can in certain situations function as a source of multipotent progenitor cells. Determining whether this is the case in human foetal eyes, however, has been difficult due to the limited number of experimental models amenable to investigating human NR growth, expansion and cell contribution. In this study, to overcome this limitation, we have successfully applied the self-organization culture approach of human ESCs to recapitulate CM development in vitro . Using induction-reversal culture combined with BMP4-triggered highly selective retinal differentiation, we demonstrated two aspects of retinal self-organization in 3D hESC culture ( Fig. 7 ): central-peripheral self-patterning of NR and self-formation of CM-like growth zones. These two aspects may be closely related: the CM-like growth zone formation occurs in the tapered portion of the NR, which resembles many of the characteristics of the peripheral domain of the embryonic NR. Thus, the presence of tissue interactions between the NR and RPE appear to foster the self-organization of stem cell niche-containing CM-like growth zones. Taken together with our previous studies [30] , [32] , we now demonstrate that self-organizing retinal culture of hESCs is capable of not only generating highly ordered epithelial structures, but also orchestrating bona fide organogenesis allowing a stem cell system to maintain and expand the developing organ in vitro . In induction-reversal culture, GSK3 and FGFR inhibitor-induced thin RPE tissue ( Rx:: Venus-dim) exhibited a transition to Rx:: Venus-strong thick NR epithelium within a few days after exposing RPE tissue to NR-differentiation medium ( Supplementary Movies 1 and 2 ). A similar induction-reversal phenomenon is also seen when only the GSK3 inhibitor was applied. However, the further addition of the FGFR inhibitor (which by itself had only weak effects if any) made RPE differentiation more complete in a relatively short period (see Methods for details). The combination of both inhibitors induces ‘all-RPE’ aggregates (with little NR-type epithelium) in >90% of aggregates of ‘induction’ culture. After removal of the inhibitors in ‘reversal’ culture, approximately three quarters of aggregates develop a NR-dominant epithelia ( Fig. 3e ; NR only+two domain). Live imaging indicated that the reappearance of NR-type epithelium in reversal culture is caused by conversion of RPE-type epithelium rather than by rapid expansion of residual NR-type epithelium in the aggregate. In addition, this ‘RPE-to-NR’ conversion, triggered only by a change in extracellular signals, can occur even after the onset of Mitf expression ( bona fide RPE marker) and the repression of Chx10 expression ( bona fide NR marker). These observations are consistent with previous studies in vivo showed a profound plasticity between the NR and RPE fates during development [41] , [42] , [54] . Interestingly, the temporal window of competence for RPE-NR reversal may be limited in our hESC culture; preliminary experiments have indicated that a longer treatment of GSK3 and FGFR inhibitors (for example, days 18–27 or 18–30, instead of days 18–24) makes RPE less responsive to reversal signals in NR-differentiation medium. This suggests that the length of RPE-specifying culture (which may deepen RPE commitment) affects the reversion efficacy. In addition, an intriguing report has described that a subpopulation of adult human RPE cells, on activation, gain competence to become multipotent stem cells [55] , suggesting that RPE cells, even in adult humans, maintain special state of epigenetic control. In future investigations, our culture method may be useful in elucidating molecular mechanisms for the stage- and species-specific control of retina transdifferentiation competence. In our hESC culture, some variation was observed in the response to the reversal trigger at the tissue level. In ~40% of aggregates, RPE and NR were co-generated (two-domain aggregates) and CM-like zones self-formed between them. In ~30% of aggregates, most of epithelia became entirely NR after reversal, whereas 25–30% of aggregates were resistant to the reversal trigger and remained RPE dominant. The cause for this heterogeneity in responsiveness is an intriguing question. We infer that it may be relevant to a ‘bistability’ control, which tends to give a ‘black-or-white’ (not grey) outcome (reviewed in ref. 56 ). In the signalling network for retinal specification ( Supplementary Fig. 2 ), RPE differentiation is promoted by Wnt signals, and, once the retinal tissue becomes RPE, it enhances local Wnt signals by inducing endogenous expression of Wnts and Mitf [57] , [58] . Conversely, NR differentiation is suppressed by Wnt signals [37] , [38] , [39] , [40] . Moreover, differentiating NR shuts off local Wnt signals by attenuating Wnt ligand production by the transcription factor Six3 (ref. 40 ) and secreting Wnt antagonists such as Dkk1 (refs 30 , 59 ). Furthermore, specification into NR and RPE is promoted and suppressed by FGF signals, respectively, which are produced by NR [41] . These multiplex regulations of mutual inhibition and autoactivation lead to a ‘bistable’ system, in which a small difference in endogenous signals could make a pivotal specification of retinal epithelium (or its local domains) into either NR or RPE. In the two-domain aggregate containing both NR and RPE, only a small portion of RPE is resistant to reversal signals promoting NR differentiation. We infer that a bias for the location of the RPE-prone domain may be related to the co-presence of nonretinal neural tissues (representing ~10% of cells; Fig. 1n,o ), which was previously shown to promote RPE differentiation within the ESC-derived optic cup [30] . Consistent with this idea, in close visual examinations of two-domain hESC aggregates after induction-reversal culture ( Fig. 3c,d ), nonpigmented Rx ::Venus − tissues (that is, nonretinal neural tissues) were not found within the continuous NR but preferentially located together with pigmented RPE. Another remaining question concerns how the boundary between RPE and NR is determined. In ‘reversal’ culture method, our preliminary observations suggest that thin RPE tissue (sometimes adjacent to nonretinal tissue) tends to resist the reversal stimuli, whereas the retinal epithelium distally (centrally) located from thin RPE tissue tends to exhibit a more rapid transition to strong Rx:: Venus-expressing thick NR epithelium. This raises a possibility that some bias in the differentiation state has already existed in RPE-like tissue before starting the reversal culture method. This hypothesis will be more rigorously tested in future studies using RPE/NR double-labelled cell lines, which might allow a more detailed observation of the dynamics of NR–RPE formation. The ‘induction-reversal culture’ method enables the co-generation of NR and RPE in hESC culture. In this continuous structure, the NR exhibits a central-peripheral polarity. With regard to morphology, a graded change in the epithelial thickness is seen along the central-peripheral (thick-to-thin) axis of hESC-derived NR. In the central portion, NR differentiation into fate-specific cells tends to be more advanced than in the peripheral portion, while immature progenitors are more prominent in the NR periphery, particularly in the tapering domain where de novo NR generation occurs. This self-formation of the central-peripheral polarity appears to correlate with the presence of RPE adjacent to the NR, since such polarity is not obvious within NR epithelia in hESC aggregates without RPE (in the latter case, the entire NR tends towards the central-NR type with regard to differentiation and thickness; Fig. 1q ). Moreover, when NR epithelium, by chance, is flanked by more than one RPE domain, a CM-like zone emerges in the NR domain next to each NR–RPE junction. It remains to be clarified whether the effect of RPE is mediated by soluble signals or spreads via planar induction. Another related question for future study is whether the effect of RPE on the central-peripheral polarity in NR is direct on the NR or secondary through the CM-like zone formation between them. In the human foetal eye, the regional difference along the central-peripheral axis is quite remarkable. For instance, the generation of morphologically recognizable photoreceptors is observed around foetal week 10 at the central-most NR region, while photoreceptor differentiation in the noncentral region occurs very gradually over the following 15 weeks and slowly proceeds in a central-peripheral pattern [44] , [60] . The central-most NR domain eventually gives rise to the fovea, in which photoreceptors are mostly cones. The generation of the fovea-like structure (a pit structure selectively expressing colour opsins and not Rhodopsin) has not been observed thus far in our culture yet, and is an intriguing and challenging topic for future study. As described in our previous report [32] , both RXR-gamma + cone precursors and Nrl + rod precursors are generated in wide domains of hESC-derived NR. Therefore, a first step towards this challenging goal may be region-selective control of cone and rod generation along the central-peripheral axis of the self-organized NR. In induction-reversal culture, the tapered peripheral end of the hESC-derived NR (sd 1), adjacent to the Mitf + domain, formed a niche for SSEA1 + stem-like cells that continuously produce progenitors. Cells in sd 1 were Ki67 + and were efficiently labelled with nucleotide analogues after 1-day of exposure, while these labels in sd 1 (showing no substantial level of apoptosis) became undetectable within 6 days, indicating that these cells are under active proliferation. sd 1, unlike sd 2, contained few fate-committed postmitotic cells and did not express CDK inhibitors (promoting cell cycle exit), suggesting that these actively proliferating cells in sd 1 were not directed to produce terminally differentiated postmitotic cells by cell cycle exit. SSEA1 + cells are also present in the CM-like zone of the mouse foetal retina. However, the strict identity of SSEA1 + cells across species could be a matter of argument. For instance, during early mouse retinal development, SSEA1 is widely expressed throughout the optic vesicle. From E13.5 onwards, SSEA1 expression is mainly seen in the peripheral NR and pigmented outer layer of the ciliary epithelium [48] . However, within the mouse peripheral NR, the nonpigmented epithelium at the peripheral end (corresponding to sd 1) is devoid of SSEA1 expression, in contrast to our finding with its expression in the CM-like tissue generated from hESCs. Since early SSEA1 expression in the mouse retina dynamically changes in a stage-specific manner [48] , a careful stage-by-stage investigation would be necessary to examine whether SSEA1 + cells in the mouse and human foetal retinae represent distinct ( albeit related) subpopulations in the growing end of the tissue. Clarke et al . recently reported the generation of ‘retinal stem-like cells’ from hESCs, but these stem-like cells may have critical differences from those generated in our study. Namely, the stem-like cells reported by Clarke et al . [53] were derived from a rare population within hESC-derived pigmented cells (stem cells from pigmented ciliary epithelial cells are also described in ref. 61 ). In contrast, the retinospheres in the present study are derived from retinal tissues from which pigmented tissues were removed. Moreover, the SSEA1 + cell population did not show obvious pigmentation in the tissue section nor by visual inspection of dissociated immunostained cells ( Supplementary Fig. 5g ; they did not show strong side scattering in FACS analysis either; not shown). Thus, the stem cell population in the CM-like zone of our hESC culture (within the Chx10 + peripheral NR) appears to be distinct from the one reported previously, which seems to be more closely related to RPE or pigmented ciliary epithelium. We infer that the 3D formation of retinal tissue with juxtaposed NR and RPE is vital for the generation of CM-type stem cells, which contribute to de novo NR extension in the peripheral direction. Regarding human retinal stem cells, another set of previous studies have suggested the presence of Müller glia-type stem cells in the marginal zone of human adult retina [19] , [62] . The similarity and difference between these adult-type cells and CM-type stem cells in our hESC culture (presumably foetal type) is another intriguing topic for future investigation. In the human foetus, the CM appears by foetal week 10 and the ciliary body formation begins at the end of the 3rd foetal month [45] . We have so far failed to observe the morphological appearance of ciliary body-like structures in our hESC culture, whereas Mitf + /Aqp1 + epithelia ( Fig. 4 ), reminiscent of ciliary epithelium, was readily generated. While the present study focused on new aspects of self-organization of hESC-derived retina, the improved culture that is introduced here also serves as an advanced protocol towards future applications of human pluripotent stem cells. First, the improved culture has enabled a more selective retinal differentiation of hESCs (>80%) by the use of timed BMP4 treatment. In our preliminary experiments, other BMPs such as BMP2, BMP7 and Gdf7 had similar inductive abilities. Moreover, unlike our and others’ previous methods, this BMP-based hESC culture does not require the xenogenic matrix protein mixture Matrigel for the 3D formation of NR. The precise mode of BMP4 action in retinal specification remains an intriguing unanswered question. Previous studies have shown that BMP signals directly suppress the expression of Foxg1, which is essential for cortical development [63] , [64] . Therefore, one interpretation may be that BMP4 treatment during the early differentiation stage in our culture prevents hESC-derived forebrain neuroepithelium from adopting the telencephalic fate and redirects it into retinal progenitors. In the early embryo, BMP signals are expressed near the anterior neural ridge and in the prechordal mesoderm, and are implicated in the patterning of rostral diencephalon of the early embryo [65] , including hypothalamic (diencephalic) induction [66] , [67] . In condition 1 of our new culture method, the continuous NR forms vesicles in apically convex manner, which resemble retinal tissues shown by Meyer et al , 2011 (ref. 27 ). The vesicles formed in our culture, however, do not undergo further morphogenesis (invagination) to form optic cup structures, since they lack RPE as the outer wall. Regarding the long-term culture, after 60 days, the NR in vesicles gradually looses its integrity and tends to accumulate neural rosettes (differentiation itself proceeds). In the induction-reversal culture combined with BMP4-induced retinal differentiation (condition 3), a portion of RPE tissue forms adjacent to NR ( Fig. 3c,d ). In this two-domain aggregate, NR is generated as a large continuous epithelium. NR can be also obtained from optic cups cultured in hESC aggregates under our previous conditions [32] . However, our new culture method has clear advantages in the reproducible generation of larger NR epithelia. First, the formation of optic cups in our previous culture was not very frequent (~10%). Second, NR epithelia in these optic cups were typically 500 μm in diameter around day 35. In contrast, NR forms as a fairly large domain (typically 1.3–1.5 mm in diameter at day 35; Fig. 3c ) with induction-reversal culture, spanning a majority of the aggregate surface, and continuous NR epithelium grows robustly (for example, typically 2 mm at day 60; Fig. 3d ). Finally, the two-domain structure of NR epithelium has a characteristic thick and transparent appearance, and its boundary to RPE can be easily recognized because of the presence of pigmented tissue adjacent to it. This simple structure may facilitate the preparation of high-purity NR tissues in large quantities (much like removing the stem ends from radishes) and may prove useful in future studies examining optic tissue transplantation, pathogenesis and drug discovery. Maintenance of hESCs hESCs (KhES-1) were used according to the hESC research guidelines of the Japanese government. hESC reporter lines ( Rx:: Venus, Rx:: AcGFP and Crx:: Venus) were generated by using Neon Transfection System (Life Technologies) [32] . hESCs were maintained on a feeder layer of MEFs inactivated by mitomycin C treatment in DMEM/F12 (Sigma; cat # D6421; suitable for 2% CO 2 culture) supplemented with 20% (vol/vol) KSR (Gibco), 2 mM glutamine, 0.1 mM nonessential amino acids (Gibco), 8 ng ml −1 recombinant human bFGF (Wako), 0.1 mM 2-mercaptoethanol, 50 U ml −1 penicillin and 50 μg ml −1 streptomycin under 2% CO 2 conditions. For passaging, hESC colonies were detached and recovered en bloc from the feeder layer by treating them with 0.25% trypsin and 1.0 mg ml −1 collagenase IV in PBS containing 20% KSR and 1 mM CaCl 2 at 37 °C for 7 min. The detached hESC clumps were broken into smaller pieces (several dozens of cells) by gentle pipetting. The passages were performed at a 1:3 to 1:5 split ratio every 3rd or 4th day. Retinal differentiation from hESCs For serum-free floating culture of embryoid body-like aggregates with quick reaggregation (SFEBq) culture, hESCs were dissociated into single cells in TrypLE Express (Gibco) containing 0.05 mg ml −1 DNase I (Roche) and 20 μM Y-27632, and quickly re-aggregated using low-cell-adhesion 96-well plates with V-bottomed conical wells (Sumilon PrimeSurface plate; Sumitomo Bakelite) in ‘differentiation medium’ (12,000 cells per well, 100 μl) supplemented with 20 μM Y-27632 (ref. 68 ) under 5% CO 2 at 37 °C. The differentiation medium is gfCDM [69] supplemented with 10% KSR, while gfCDM contains 45% Iscove’s modified Dulbecco’s medium (IMDM, Gibco), 45% Hams F12 (F12, Gibco), Glutamax, 1% chemically defined lipid concentrate (Gibco), monothioglycerol (450 μM, Sigma), 100 U ml −1 penicillin and 100 μg ml −1 streptomycin (Gibco). Defining the day on which the SFEBq culture was started as day 0, recombinant human BMP4 (R&D) was added to the culture to the final 1.5 nM (55 ng/ml) on day 6, and its concentration was diluted into half by half medium change every 3rd day. The addition of BMP4, started on day 3 and day 6, induced Rx + NR epithelium at day 18 with similar efficiency. The number of initial plating of cells (12,000 cells per well) was optimized (in both efficiency and size), but Rx + NR epithelium was also achieved using 9,000 cells per well. To establish NR-differentiation culture from hESCs without the use of Matrigel, we examined the effects of the following signal modulators on the induction of Rx:: Venus + cells at various doses and time points: BMP agonists/antagonists (BMP4, dorsomorphin), Wnt agonists/antagonists (Wnt3a, IWR1e), Shh agonists/antagonists (SAG, cyclopamine) and FGF agonists/antagonists (FGF2, SU5402). Among them, the addition of BMP4 at low concentrations during early phases of SFEBq culture (day 3 or day 6) proved to most effectively induce Rx:: Venus + retinal epithelium on day 24. Long-term NR culture NR epithelium was subjected to long-term culture under the following conditions: on day 18, NR-containing aggregates were transferred from a 96-well plate to a 9-cm Petri dish (noncell adhesive; Sumitomo Bakelite) and further cultured in suspension (60 aggregates/9-cm dish for days 18–50; 30 aggregates after day 50) under 40% O 2 /5% CO 2 conditions in ‘NR-differentiation medium’ containing DMEM/F12-Glutamax medium (Gibco), 1% N2 supplement (Gibco), 10% foetal bovine serum (FBS), 0.5 μM retinoic acid (Sigma), 0.1 mM taurine (Sigma), 0.25 μg ml −1 Fungizone (Gibco), 100 U ml −1 penicillin and 100 μg ml −1 streptomycin. NR tissues continuously grew under these conditions for the next several weeks, at least. RPE tissues grew slowly compared with NR tissues. Induction-reversal culture To induce CM-like tissues within NR, NR epithelium generated from hESCs was subjected to two-step ‘induction-reversal’ culture under the following conditions. For the ‘induction’ culture, NR-containing aggregates generated from hESCs on day 18 were transferred from a 96-well plate to a 9-cm Petri dish (noncell adhesive), and further cultured in suspension for 4–6 days under 5% CO 2 conditions in DMEM/F12-Glutamax medium containing 1% N2 supplement, 3 μM CHIR99021 (GSK3 inhibitor; Stemgent), 100 U ml −1 penicillin and 100 μg ml −1 streptomycin. The addition of 5 μM SU5402 (FGFR inhibitor; Sigma) treatment to this induction medium increased efficiency and reproducibility of RPE induction and formation of CM-like tissues after the reversal culture, while CHIR99021 treatment without SU5402 tended to give higher variations in the level of RPE induction. For the ‘reversal’ culture, the floating aggregates with RPE-like thin epithelium ( Fig. 2b,c ) were cultured in suspension under 40% O 2 /5% CO 2 conditions in NR-differentiation medium (described above). On day 50, two-domain aggregates with CM-like tissues formed and they were further cultured in NR-differentiation medium. Two-domain aggregates with CM-like tissues stably grew in long-term culture. For the reversal culture, the addition of FBS is essential and its depletion from the reversal culture medium substantially decreased NR differentiation. CM-like tissues could be also generated by the induction-reversal culture using NR epithelia obtained by our previous method using Matrigel [32] . CM-like tissues generated by using Matrigel and induction-reversal culture were similar to those generated by using induction-reversal culture with BMP4 treatment, as judged by CM marker expression and morphology (data not shown). NR epithelia generated with Matrigel tended to be more sensitive to RPE-induction medium than BMP4-induced NR and more reproducibly underwent RPE differentiation in medium containing CHIR99021. Both our previous method [32] (Matrigel based) and new method (BMP treatment) showed a similar time course of differentiation: Brn3b + cells (~d28), Crx + cells (~d35), Recoverin + (~d45), RXRG + cells (~d60), NRL + cells (~d100), S-opsin + cells (~d130) and Rhodopsin + cells (weak expression, ~d130). CRALBP + or GFAP + cells (Muller glia) and PKC-alpha + cells (bipolar cells) were not yet detected (~d140). When we applied the ‘induction-reversal’ methods, differentiation of these markers tended to be delayed by several days (corresponding to the time for RPE-induction phase). NR progenitors, generated by BMP treatment with ‘induction-reversal’ method, differentiated into Crx + photoreceptors by DAPT (Sigma) treatment for 7 days ( Supplementary Fig. 7 ) as described previously [32] . Floating aggregates and retinospheres were analyzed with a fluorescence microscope (KEYENCE, BIOREVO). Retinosphere formation and differentiation For sphere formation assays, aggregates with CM-like tissues (day 60–90) were manually dissected into CM-like tissues (tapering NR without pigmented RPE tissue) and nonmarginal NR tissues (nontapering central NR) using fine forceps under stereo microscope (Olympus, SZX16). After digestion in papain (Sumitomo Bakelite) at 37 °C for 30 min, both tissues were gently dissociated into single cells by pipetting. Dissociated single cells were plated on 96-well flat bottom plates (MPC coated; Nunc) at a density of 1,000–3,000 cells per well (0.5–1.5 × 10 4 cells per ml) and cultured for 7 to 14 days in ‘retinosphere medium’ containing DMEM/F12-Glutamax medium, 2% B27 supplement (without vitamin A; Gibco), 20 ng ml −1 human bFGF, 20 ng ml −1 human EGF (R&D), 5 μg ml −1 heparin (Sigma), 0.25 μg ml −1 Fungizone, 100 U ml −1 penicillin and 100 μg ml −1 streptomycin. For secondary sphere formation assay, primary spheres were dissociated by using papain and cultured in retinosphere medium. For retinosphere differentiation assays, retinospheres were plated on poly- D -lysine (Sigma) and Laminin (Invitrogen)-coated dishes (five spheres per cm 2 ) and cultured in DMEM/F12-Glutamax medium, 2% B27 supplement, 20 ng ml −1 human bFGF, 5 μ ml −1 heparin, 0.25 μg ml −1 Fungizone, 100 U ml −1 penicillin and 100 μg ml −1 streptomycin for 2 days. The cells were further cultured for 10–14 days in retinosphere differentiation medium, containing DMEM/F12-Glutamax medium, 1% N2 supplement, 10% FBS, 0.5 μM retinoic acid, 0.1 mM taurine, 10 μM DAPT, 0.25 μg ml −1 Fungizone, 100 U ml −1 penicillin and 100 μg ml −1 streptomycin. FACS and MACS For FACS analysis ( Fig. 1o,p ), cells (from 24 aggregates per each sample, n =3) were dissociated into single cells using Accumax (Innovative Cell Technologies) and analyzed by using FACSAria with FACSDiva software (Becton Dickinson). For FACS or MACS sorting, dissected tissues were dissociated into single cells by using papain (described above), and then immunostained with an SSEA1-APC antibody (Becton Dickinson; for FACS) or SSEA1-MicroBeads antibody (Miltenyi Biotec; for MACS) at 4 °C for 15–30 min. For FACS, cells were sorted into Rx:: Venus-positive/SSEA1-APC + fraction and Rx:: Venus-positive/SSEA1-APC − fractions using FACSAria with the FACSDiva software. For MACS, cells were sorted into SSEA1 + or SSEA1 − fractions using autoMACS Pro (Miltenyi Biotec) according to manufacturer’s instruction. BrdU and EdU labelling BrdU and EdU labelling were performed at different time courses as indicated. NR+RPE-containing two-domain aggregates were cultured in NR-differentiation medium in the presence of BrdU (5 μg ml −1 , 16 μM; Sigma) for 24 h. Then, aggregates were washed with medium and cultured in the absence of BrdU. For BrdU and EdU double labelling assays, aggregates were further cultured with EdU (10 μM; Molecular Probes) in NR-differentiation medium, washed and cultured in the absence of EdU. Aggregates were fixed at 4 °C in 4% paraformaldehyde in PBS for 15 min. BrdU was detected by immunostaining. EdU was detected by the Click-it assay according to the manufacturer's protocol. Immunohistochemistry Immunohistochemistry was performed as described [30] . Frozen sections were treated with or without heat-based antigen retrieval in Target Retrieval solution (15 min at 105 °C; DAKO). Primary antibodies used in this study are described as follows: GFP (rabbit/1:500/MBL), (rat/1:500/Nacalai) or (mouse/1:1,000/Invitrogen), Pax6 (rabbit/1:200/Covance), Chx10 (goat/1:100/Santa Cruz) or (sheep/1:500/Exalpha), Mitf (mouse/1:500/Exalpha), Sox2 (goat/1:500/Santa Cruz), N-cadherin (Mouse/1:500/BD), phospho-Histone H3 (rabbit/1:500/Upstate), aPKC (rabbit/1:100/Santa Cruz), Laminin (mouse/BD/1:1,000), Collagen IV (rabbit/ARP/1:1,000), Entactin (rat/Abcam/1:1,000), TuJ1 (mouse/Covance/1:500), Blimp1 (rat/1:100/Santa Cruz), Brn3b (goat/1:100/Santa Cruz; C-13), Ptf1a (armenian hamster/1:3; kind gift from Dr Yuichi Ono, KAN Institute), Recoverin (rabbit/1:500/Chemicon), Calbindin (rabbit/1:500/Millipore), Calretinin (rabbit/1:1,000/Chemicon), S-opsin (rabbit/1:500/Millipore), Rhodopsin (mouse/1:1,000/Sigma; RET-P1), NRL (goat/1:500/R&D), RXR-gamma (rabbit/1:500/Spring Bioscience), Cleaved Caspase 3 (rabbit/1:500/CST), Ki67 (mouse/1:200/BD) or (rabbit/1:200/Novocastra), p27 (C-19; rabbit/1:500/Santa Cruz), p57 (rabbit/1:500/Sigma), p21 (mouse/1:100/Santa Cruz), BrdU (mouse/1:50/BD), SSEA1 (mouse IgM/1:100/Chemicon), Aqp1 (rabbit/1:500/Millipore), Rdh10 (rabbit/1:200/Proteintech), Otx1 (mouse/1:1,000/DSHB), Crx (rabbit/1:200/raised in-house), and Zic1 (rabbit/1:20,000/raised in-house). The antiserum against Crx was raised in rabbits against mixed synthetic peptides of 5′- CLEFKDPTGTWKFTYNPMDPLDYKDQSAWKFQIL -3′ (Crx 266–299) and 5′- KARPAKRKAGTSPRPSTDVCPDPLGISDSY -3′ (Crx 113–143) and was affinity purified. Counter nuclear staining was performed with 4',6-diamidino-2-phenylindole (DAPI; Nacalai). Stained sections were analyzed with an LSM710 confocal microscope (Zeiss). Live imaging of retinal epithelium Aggregates with RPE-like thin epithelium on day 24 were embedded in undiluted Matrigel on a 3.5-cm glass-bottom dish (Matsunami) and immersed in either ‘RPE-induction medium’ (containing DMEM/F12, 1% N2 supplement, 1% FBS and 3 μM CHIR99021; condition 2) or NR-differentiation medium (described above; condition 3). Live imaging was performed as described [30] using a specially assembled inverted spinning-disc confocal microscope combined with a full-sized CO 2 /O 2 incubator. Images were analyzed with the MetaMorph software (Molecular Devices) and Image-J. Similar results were obtained in six aggregates in three independent experiments. Animals Pregnant ICR mice were obtained from Japan SLC (Japan). The day of the vaginal plug detection was designated as embryonic day 0.5 (E0.5). All animal experiments were performed in compliance with the Guidelines for Use of Laboratory Animals of RIKEN. Statistical analysis Statistical tests were performed with the PRISM software (GraphPad, version 5). Statistical significance was tested with Student’s t -test (parametric) or Mann–Whitney’s test (nonparametric) for two-group comparisons and with analysis of variance followed by post-hoc Tukey’s test for multi-group comparisons. How to cite this article: Kuwahara, A. et al . Generation of a ciliary margin-like stem cell niche from self-organizing human retinal tissue. Nat. Commun. 6:6286 doi: 10.1038/ncomms7286 (2015).